Whole-genome sequencing reveals untapped genetic potential in Africa’s indigenous cereal crop sorghum Sorghum is a food and feed cereal crop adapted to heat and drought and a staple for 500 million of the world’s poorest people. Its small diploid genome and phenotypic diversity make it an ideal C 4 grass model as a complement to C 3 rice. Here we present high coverage (16–45 × ) resequenced genomes of 44 sorghum lines representing the primary gene pool and spanning dimensions of geographic origin, end-use and taxonomic group. We also report the first resequenced genome of S. propinquum , identifying 8 M high-quality SNPs, 1.9 M indels and specific gene loss and gain events in S. bicolor. We observe strong racial structure and a complex domestication history involving at least two distinct domestication events. These assembled genomes enable the leveraging of existing cereal functional genomics data against the novel diversity available in sorghum, providing an unmatched resource for the genetic improvement of sorghum and other grass species. Increasing global demand for food, driven by population growth and rising affluence, will impose severe challenges on the agricultural and social systems supporting the world’s poorest people [1] . The challenges facing these people will be further exacerbated by decreasing vital resources for agriculture and the inequitable negative impacts of climate change [2] . Input-intensive crops will fall into disfavour, particularly in agricultural systems that are resource-poor [3] . Sorghum, already a staple for half a billion people, and tolerant of low input levels [4] , will become increasingly critical in these systems [5] , particularly in Sub-Saharan Africa. Globally, sorghum is also an important source of animal feed and forage, an emerging biofuel crop and model for C 4 grasses particularly genetically complex sugarcane [6] . The full exploitation of sorghum’s potential requires an understanding of genetic diversity at the genomic sequence level. Cultivated grain sorghum ( Sorghum bicolor subsp. bicolor ) is a domesticate of the wild progenitor S. bicolor subsp. verticilliflorum [7] . It is hypothesised that sorghum, the only globally important cereal from Africa, was first domesticated in Ethiopia and Sudan >8,000 years ago [8] . Subsequently, sorghum spread to west and southern Africa and into Asia as far east as China. Stable weedy hybrids between cultivated sorghum and wild types are known as S. bicolor subsp. drummondii . Notably, these three subspecies appear to be sympatric in most areas that sorghum is cultivated and there is ample evidence for gene flow in both directions. Although bidirectional gene flow is not unique among major crops plants [9] , sorghum is the only major cereal where the wild/weedy relatives have followed the cultivated species by inadvertent introduction from Africa into the Americas, Asia and Australia; hence, crop–wild–crop gene flow occurs almost everywhere sorghum is cultivated. Here we present genomic sequences of 44 sorghum accessions spanning the dimensions of geographic origin, crop management and subgroup/race at mid–high coverage levels. Our findings indicate that sorghum offers unique and underdeveloped genetic resources amongst the major cereals. We observed strong racial structure and complex domestication events. Foremost, we find that modern cultivated sorghum is derived from a limited sample of racial variation. A great untapped pool of diversity exists not only in the other races of S. bicolor but also in the allopatric Asian species, S. propinquum. This diversity is easily accessed in breeding endeavours because of well-documented interfertility among races and beyond other sorghum species. These sequences and associated data represent an unmatched resource for research into the genetic improvement of this cereal crop to meet future demands. Sequencing and variation calling We selected 44 accessions to represent all major races of cultivated S. bicolor , in addition to its progenitors and S. propinquum ( Supplementary Fig. S1 ; Supplementary Data 1 ). Among these lines, 18 are considered to be landraces, 17 are improved inbreds and 7 are wild and weedy sorghums ( Supplementary Fig. S2 ). Recent studies [10] , [11] have indicated that the guinea-margaritiferums are highly divergent from other cultivated S. bicolor races and possibly represent a separate domestication event. Consequently the guinea-margaritiferum genotypes were separated into a distinct group. Resequencing of the 44 sorghum genotypes yielded 7.97 billion 90-bp paired-end reads, which comprised 717 Gb of high-quality raw data ( Supplementary Data 1 ; Supplementary Fig. S3 ). We combined this with 27 Gb (three genotypes) of publically available raw data [12] . Sequence reads were aligned to the sorghum reference genome, which has an effective genome length of ~700 Mb [6] , using BWA software [13] . The mapping rate in different accessions varied from 78% to 99%, averaging 97% in S. bicolor lines, 89% among wild relatives. Observed differences in mapping rates may be due to divergence between the sequenced genotypes and the reference genome, BTx623. The average final effective mapping depth achieved was ~22 × per line, ranging from 16 × to 45 × . 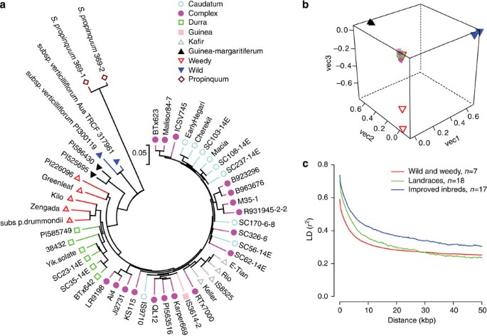Figure 1: Analysis of the phylogenetic relationship and LD decay of sorghum. (a) A neighbor-joining tree constructed using SNP data. (b) Principal component analysis of sorghum accessions. (c) LD decay determined by squared correlations of allele frequencies (r2) against distance between polymorphic sites in wild and weedy sorghum genotypes (red), landraces (green) and improved inbreds (blue). Using a conservative quality filter pipeline (see Supplementary Methods ), we identified 4,946,038 SNPs genome-wide in S. bicolor alone ( Table 1 ), with 809,460 SNPs in the 29,346 high-confidence filtered gene set (FGS). The 1,982,971 insertions and deletions (indels) identified ranged from 1–66 bp in length. Targeted sequencing of 2,917 predicted base positions validated 99.85% of SNPs and indels ( Supplementary Data 2, 3 ). Further, whole-genome de novo assembly of representative lines showed a common position SNP calling accuracy rate of 99.72% ( Supplementary Data 4, 5 ). To our knowledge, this represents the largest high-quality SNP and indel data set obtained in sorghum. Table 1 Summary SNP statistics in Sorghum bicolor genotypes. Full size table Of the 4.9 million high-quality SNPs, most (83%) were located in intergenic regions, with an average of 4.5% (ranging from 4.1% for landraces to 5.3% for improved inbreds) located in coding sequences ( Supplementary Table S1 ; Supplementary Fig. S4 ; Supplementary Data 6 ). Coding regions displayed lower diversity levels relative to intron and UTR sequences ( Supplementary Fig. S5 ). Among coding regions, there were 112,255 synonymous and 112,108 non-synonymous SNPs, resulting in a non-synonymous-to-synonymous substitution ratio of 1 and a corresponding overall Ka/Ks value of 0.441 ( Supplementary Tables S2,S3 ). Previous studies in sorghum [14] , [15] have also found fewer non-synonymous than synonymous substitutions. In comparison to other genome-wide studies, sorghum’s non-synonymous to synonymous substitution ratio is within the range reported for other plant species (soybean 1.37 (ref. 16 ), rice 1.2 (ref. 17 ), Arabidopsis 0.83 (ref. 18 )). Non-synonymous to synonymous substitution rates varied genome-wide with heterochromatic regions having higher Ka/Ks values (euchromatin: 0.423; heterochromatin: 0.502), consistent with soybean [19] ( Supplementary Table S4 ). The average Ks value in the heterochromatin (0.0169) was lower than in euchromatin (0.0201), indicating a slower rate of evolution in heterchromatic regions. Little difference was observed between the Ka values in the heterochromatin (0.0058) and euchromatin (0.0054), which could suggest that both genomic regions experience similar levels of selective constraints. The non-synonymous to synonymous substitution ratios in duplicated genes (0.779) was marginally lower than the whole-genome average (0.999) suggesting that non-synonymous changes have not accumulated more rapidly in recently duplicated genes, in agreement with a recent report in soybean [16] ( Supplementary Fig. S6 ). A total of 1,982,971 small-to-medium length indels were identified with nearly equal numbers of insertions (872,080) and deletions (1,110,891) ( Supplementary Tables S5,S6 ). Most indels (86%) were small (1–6 bp), with only 2.5% greater than 20 bp in length ( Supplementary Fig. S7 ). The majority (83%) were located in intergenic regions, with only 1.5% (29,697) located in coding regions, of which 35% resulted in frame-shift mutations. In contrast, indels with lengths that were multiples of three were less prevalent in non-coding regions (an average of 18.3% versus 63%). Based on coverage depth and a recently published event-testing algorithm [20] , 120,929 copy number variations (CNVs) were identified, 16% of which occurred in genic regions ( Supplementary Fig. S8 ). In total, 28% of sorghum genes in the FGS had CNVs, of which 1,379 (16%) were duplicated genes. Of these, 224 were in common across all three groups and were enriched for auxin responsive proteins and zinc finger proteins, in line with a previous sorghum study [12] ( Supplementary Fig. S9 ). The number of SNPs was higher in wild and weedy sorghum genotypes than in landraces and improved inbreds ( Table 1 ; Supplementary Fig. S10 ) Wild-specific alleles (34%) were more abundant than improved inbred specific alleles (8%) and landrace specific alleles (18%). Similarly, the average total number of SNPs and indels per genotype was lowest in the improved inbreds and highest in the wild species, equating to an average of 1 SNP per 1,543 bp, 1,282 bp and 763 bp for the improved inbreds, landraces and wild and weedy groups, respectively. Guinea-margaritiferum genotypes had approximately twice the SNP density of the landrace group (1 SNP per 691 bp versus 1 SNP per 1,282 bp, respectively). The lower level of diversity in the improved inbreds was also detected using θ π and θ w ( Table 1 ) and was significantly lower ( P <2.2 e −16 by paired t -test) compared with both the landraces and wild and weedy genotypes ( Supplementary Fig. S11 ). The apparent rates of heterozygous SNPs were also lower in the improved inbred lines in comparison to the landraces, guinea-margaritiferums and wild and weedy genotypes ( Supplementary Fig. S12a ). However, distinct heterozygous features were identified genome-wide, which corresponded to CNVs, suggesting that a significant proportion of the apparent heterozygous SNPs are infact paralogous sequence variants ( P =0.001199 by χ 2 test; Supplementary Fig. S12b ), defining regions collapsed in the reference genome, as also identified previously [21] . Estimated diversity levels were comparable to previous sorghum studies [14] , [15] , [22] , [23] demonstrating that wild sorghum is more diverse than improved inbreds and indicating genetic bottleneck events have occurred during both domestication and improvement. These results underscore the significance of wild sorghum germplasm as a valuable and untapped resource for sorghum improvement and that unique genetic features of the guinea-margaritiferum genotypes may be useful for improvement. Divergence between wild and cultivated sorghums The Asian diploid S. propinquum (2 n =2 × =20) is divergent from other resequenced sorghums ( Fig. 1 ), with 22% of S. propinquum reads unmapped to S. bicolor . S. propinquum alleles were the most divergent at all loci and possessed the majority of gene gain/loss events observed. Evidence for gene flow from S. propinquum into cultivated sorghums is absent within our data; thus, as a member of the primary gene pool, the interfertile S. propinquum remains underutilised. Figure 1: Analysis of the phylogenetic relationship and LD decay of sorghum. ( a ) A neighbor-joining tree constructed using SNP data. ( b ) Principal component analysis of sorghum accessions. ( c ) LD decay determined by squared correlations of allele frequencies ( r 2 ) against distance between polymorphic sites in wild and weedy sorghum genotypes (red), landraces (green) and improved inbreds (blue). Full size image Recent hypotheses [11] , [23] , [24] proposed that guinea-margaritiferums are the result of a second and more recent domestication in West Africa. Guinea-margaritiferums are not only phenotypically distinct from the other guinea types [11] , but appear as intermediates between cultivated sorghum and the wild S. bicolor subsp. verticilliflorum in all of our phylogenetic analyses ( Fig. 1a ). This is in line with the recent study of 971 sorghum accessions based on genotyping-by-sequencing (GBS) data [23] , which observed that the guinea-margaritiferums types formed a separate cluster along with wild genotypes from western Africa, supporting a possible independent domestication. Principal components analysis ( Fig. 1b ) shows that the cultivated and weedy genotypes cluster together, with S. bicolor subsp. verticilliflorum separating on principal component 1 followed by guinea-margaritiferums on principal component 2, explaining 55% of the variation. The guinea-margaritiferums separate in structure plots from the wild progenitor at K =5 ( Supplementary Fig. S13 ). Despite origins in different countries, the guinea-margaritiferums in this study have distinct allelic variants at major domestication and grain quality loci including TeosinteBranched1 ( Tb1 ), GrainSize3 ( GS3 ) and starch synthase genes ( Fig. 2 ). The West African origins of guinea-margaritiferums, where poor soils and unreliable rainfall are noteworthy, suggest an extremely valuable genetic resource for low soil pH and toxic aluminium tolerance [25] . 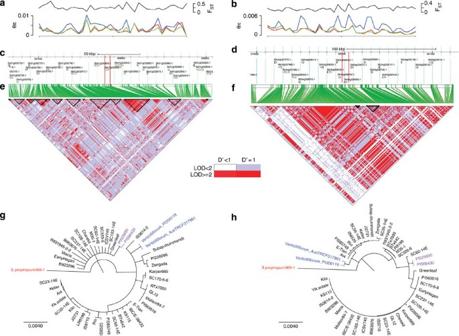Figure 2: Signatures of selection in two genomic regions. (a,b) Diversity (θπ) (wild and weedy group in red; landraces in blue, improved inbreds in green) andFSTvalues (black line) in 10-kb intervals. (c,d) Predicted gene models in genomic regions with candidate genes under selection highlighted, Sb01g032830 (SbGS3) and Sb04g028060 (SSIIb), respectively. (e,f) LD blocks around candidate genes under selection. Red and white spots indicate strong (r2=1) and weak (r2=0) LD, respectively. (g,h) Gene trees forGS3andSSIIb, respectively. Figure 2: Signatures of selection in two genomic regions. ( a , b ) Diversity ( θ π) (wild and weedy group in red; landraces in blue, improved inbreds in green) and F ST values (black line) in 10-kb intervals. ( c , d ) Predicted gene models in genomic regions with candidate genes under selection highlighted, Sb01g032830 ( SbGS3 ) and Sb04g028060 ( SSIIb ), respectively. ( e , f ) LD blocks around candidate genes under selection. Red and white spots indicate strong ( r 2 =1) and weak ( r 2 =0) LD, respectively. ( g , h ) Gene trees for GS3 and SSIIb , respectively. Full size image Tajima’s D statistics obtained from our data are in agreement with previously reported values [22] , and support a recent population bottleneck. Estimates for a time of domestication are within the range of archaeological findings of sorghum grain in storage vessels dating back 8,000 years. As a result of domestication, linkage disequilibrium (LD) increased markedly in improved sorghum. The average distance over which LD decays to half of its maximum value in sorghum is between 19.7 kb and 10.3 kb for the improved inbreds and landraces respectively and extended to background levels within ~150 kb ( Fig. 1c ; Supplementary Fig. S14 ). These are intermediate to values recently reported for rice [26] (65 kb for subsp . indica and 200 kb for subsp . japonica ), soybean [16] (~150 kb and 75 kb for cultivated and wild respectively) and maize [27] (<1 kb) and very similar to recent LD estimates in sorghum [23] based on GBS data across 971 accessions. The LD decay estimates based on the resequencing and GBS data in sorghum are higher than previous estimates [28] , [29] in sorghum, likely due to the low genome coverage of markers and fewer genotypes in earlier studies. Regions of the genome under selection Human-mediated selection has frequently resulted in crops that have a similar suite of agricultural characteristics (the domestication syndrome), low levels of genetic variation and skewed allele frequency spectra, for example, maize [30] , rice [26] and soybean [16] . Wild sorghums provide a resource to study the impact of human selection on the patterns of genetic variability in comparison to cultivated germplasm. To detect selective sweeps, driven by both domestication and improvement, we sought to identify genomic regions with elevated differentiation between wild, landrace and improved groups. Additionally we sought low nucleotide diversity and skewed allele frequency spectra in non-overlapping windows of 10 kb along the entire genome for each group, and for the annotated regions of each gene in the FGS ( Fig. 3 ; Supplementary Figs S15–S24 ). Adjacent windows meeting these criteria were grouped into ‘features’, each likely representing the effect of a single selective sweep. 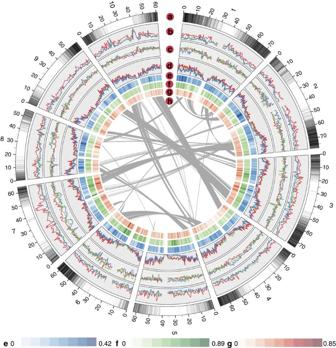Figure 3: Summary of sorghum resequencing data. Concentric circles show the different features that were drawn using the Circos program57. The 10 chromosomes are portrayed along the perimeter of each circle. (a) Gene content density distribution. (b) Genomic diversity (θπ) of wild and weedy genotypes (red), landraces (green) and improved inbreds (blue). (c) Tajima’sDof wild and weedy genotypes (red), landraces (green) and improved inbreds (blue). (d) Number of SNPs in wild and weedy genotypes (red), landraces (green) and improved inbreds (blue). (e)FSTvalues of improved inbreds versus landraces. (f)FSTvalues of improved inbreds versus wild and weedy genotypes. (g)FSTvalues of landraces versus wild and weedy genotypes. (h) A graphical view of duplicated annotated genes is indicated by connections between segments. Figure 3: Summary of sorghum resequencing data. Concentric circles show the different features that were drawn using the Circos program [57] . The 10 chromosomes are portrayed along the perimeter of each circle. ( a ) Gene content density distribution. ( b ) Genomic diversity ( θ π) of wild and weedy genotypes (red), landraces (green) and improved inbreds (blue). ( c ) Tajima’s D of wild and weedy genotypes (red), landraces (green) and improved inbreds (blue). ( d ) Number of SNPs in wild and weedy genotypes (red), landraces (green) and improved inbreds (blue). ( e ) F ST values of improved inbreds versus landraces. ( f ) F ST values of improved inbreds versus wild and weedy genotypes. ( g ) F ST values of landraces versus wild and weedy genotypes. ( h ) A graphical view of duplicated annotated genes is indicated by connections between segments. Full size image Overall, we identified 725 candidate genes for domestication and/or improvement using the gene-based population summary statistics ( Supplementary Data 7–9 ). Similarly, we identified 1,228 10 kb+ candidate domestication and/or improvement features ( Supplementary Data 10 ). As shown previously in maize [30] , improvement features had smaller average sizes than domestication features and contained fewer genes ( Supplementary Table S7 ). A number of candidate genes for domestication and/or improvement were identified within these features. Only a small proportion of the identified candidate genes were in common based on the two different scales used ( Supplementary Fig. S25 ). We found that 33% of the candidate domestication genes (285) showed additional evidence of selection during improvement, signifying that a subset of domestication loci may contribute to phenotypes associated with continued agronomic performance. To validate whether the domestication and improvement candidates showed patterns of genetic variation consistent with positive selection we used the mlHKA test [31] . A model of directional selection best explained the patterns of polymorphism to divergence at 422 candidate genes for domestication and improvement relative to 10 neutral loci (mean log likelihood ratio test statistic=2,862; P =0 for all comparisons; Supplementary Table S8 ). Overall, 50% (621) of the identified features associated with selective sweeps contained zero predicted genes, potentially implicating a role for regulatory variation in crop evolution. A further 259 features were fixed between groups ( Supplementary Table S9 ). Invariant features were smaller on average than features under selection and contained fewer genes; overall, 75% (193) of invariant features did not contain genes. This again implicates non-genic regulatory elements in the evolution of cultivated sorghum and also raises the possibility that many of these regions may be in LD with a selected genic region (genetic hitchhiking). Of the 814 ‘zero gene’ invariant features or features under selection, only 8.5% (70) were in LD (within 20 kb) with candidate genes for domestication and improvement, suggesting that hitchhiking may not be important for features without genes. Additionally, no previously described miRNA sequences [6] , [32] were located in these regions. In total, we found 14% of the FGS to be invariant within and among the three groups ( Supplementary Fig. S26 and Supplementary Data 11–13 ). As expected, the proportion of invariant genes specific to the improved inbreds was the largest (22%) in comparison to the landraces (15.8%) and the wild and weedy group (10.5%). Duplicated genes were less likely to be invariant. Generally, we found that genes with essential biological functions, for example, organ development and reproduction, were enriched in the invariant class across all three groups ( Supplementary Figs S27–S30 ). Interestingly, 91 genes were fixed across all three groups, but were polymorphic in the guinea-margaritiferums. These were found to include genes associated with lipid biosynthesis, including serine palmitoyltransferase (Sb03g039400) involved with sphingolipid biosynthesis, which has been postulated to have a role in signal transduction, host–pathogen interactions and stress responses [33] . Of the 91 genes, half (45) had either large-effect SNP (LE-SNPs) or non-synonymous mutations in the guinea-margaritiferums, including SbIAA26 , an auxin responsive protein (Sb10g023210) and Sb03g036700, a drought-inducible protein, potentially involved in novel functionality specific to the guinea-margaritiferums. We found only three invariant genes in common between sorghum and maize [34] , [35] ( Supplementary Fig. S31 ), one of which (Sb04g024055, SbXRCC3 ) has a crucial role in recombination [36] . Approximately half of the candidate genes under selection (55.5%) and invariant genes (48.3%) colocated with previously identified domestication loci in sorghum and other cereals, including the well known domestication genes, Tb1 and ba1 (ref. 37 ). The regions embedding both Tb1 and ba1 show a large reduction in diversity around these genes in the cultivated lines compared with the wild and weedy genotypes ( Supplementary Figs S32,S33 ), and the gene trees are also indicative of a selective sweep, with star-like branches in the cultivars but long branches in wild sorghum. Strong signatures of selective sweeps were identified around other key genes including dep1 , a gene which enhances grain yield in rice [38] , Psy1 , a gene controlling grain colour [39] and Bif1 , a gene associated with plant architecture in maize [40] ( Supplementary Figs S34–S36 ). Additionally, strong signatures of selective sweeps were identified around key major effect genes [41] associated with domestication traits including grain-related traits, plant colour, height and maturity, for example, Ma 1 and dw 2 on SBI-06, dw 3 on SBI-07 and Ma 4 on SBI-10. Subregions that have very high F ST values may prove useful both in dissecting existing QTL and major effect genes and identifying novel candidate genes for these traits ( Supplementary Fig. S37 ). For example, the major latex protein family member, Sb07g023210, is found under the F ST peak within the genomic region controlling the grain colour gene ( I ), which has been associated with fruit and flower development [42] . To assess possible gene functions targeted by both improvement and domestication, we used gene function annotation [43] , [44] ( Supplementary Figs S38–S40 ). Gene families related to auxin responsiveness, involved in biotic and abiotic stress responses, were enriched in the candidate improvement and domestication genes ( P =0.001368 by χ 2 test), including members of the GH3, SAUR and IAA families. Improvement and domestication candidate genes were also enriched for the GO-SLIM category adenyl ribonucleotide ( P =0.000997 by χ 2 test) and included the sorghum ortholog of MLH3 (Sb02g032160), a gene required for cross-over formation during meiosis [36] . A proportion (21.6%) of the candidate genes under selection have yet to be functionally annotated. The candidate domestication and improvement genes provide opportunities to further enhance existing knowledge and to rapidly identify genes with agronomic significance in sorghum. Deleterious mutations and gene content variation LE-SNPs, which affect intron splicing as well as polypeptide chain initiation and termination, totalled 6,940 variations in 2,273 genes across the wild and weedy, landrace and improved inbred lines ( Supplementary Fig. S41 ; Supplementary Table S10 ). This represents 7.7% of the sorghum genes affected and is intermediate between A. thaliana [18] (6.1%) and soybean [16] (10%) ( Supplementary Data 14 ). A further 51,135 frame-shift indels were present in 5,749 genes, of which 17% were unique to S. propinquum . These variations, which alter the primary amino-acid sequence, were under-represented in genes from the cellular component GO-SLIM category, and included the known domestication loci Rc (pericarp colour [45] ) and su1 (starch biosynthesis [37] ; Supplementary Fig. S42 ). Deletions in SbRc were unique to the guinea-margaritiferum accessions while members of the improved inbred group were affected by a specific deletion in Sbsu1 . The guinea-margaritiferum accessions had, on average, five-fold more LE-SNPs compared with members of the improved inbred and landrace groups and the most frame-shifting indels of all the accessions ( Supplementary Fig. S43 ). A functional analysis of LE-SNPs and frame-shifting indels unique to the guinea-margaritiferums genotypes revealed multigene family members implicated in biotic and abiotic stress, including orthologs of Arabidopsis BTB/POZ-MATH 1 and 2 ( BPM1 and BPM2 ), and four pathogen response-related proteins. These results highlight the value of the unique genetic features within the guinea-margaritiferum accessions ( Supplementary Fig. S44 ). Larger deletions, which encompassed over 50% of the annotated gene sequence, were identified by examining read depth at 100 bp resolution across the FGS gene models and in the 1 kb flanking each end. These large deletions were identified in 757 genes ( Supplementary Data 15 ) and a subset validated by PCR ( Supplementary Figs S45–46 ). Of the 757 gene loss events, 12.5% were unique to the landraces and 8.2% to the wild and weedy genotypes ( Supplementary Fig. S47 ). Nine gene-loss events were unique to the guinea-margaritiferums and include a GRAS family transcription factor member (Sb05g026260), thought to be involved with developmental processes [46] . Notably, amongst the genes present in the guinea-margaritiferums but with gene deletion events in the other S. bicolor genotypes were domestication genes related to tillering (for example, Tb1 ; Sb01g010690) and maturity (for example, SbFRI ; Sb01g0010300). These variations may be indicative of the different selective forces applied to wild and cultivated sorghum given their different habitats and breeding practices. Such gene-loss events may contribute to heterosis and therefore be important in breeding programs. Novel genes were identified based on sequence homology to plant reference proteins using predicted gene models derived from the de novo assembly of unmapped reads and verified by PCR ( Supplementary Fig. S48 ). In keeping with recent observations in rice [26] our conservative set of 101 novel genes was generally shorter in length (average of 1,258 bp) than those mapped to the genome (averaging 1,709 bp), indicating that some of the novel genes are not intact genes and some may be pseudogenes ( Supplementary Table S11 ). The wild and weedy genotypes had 7.2% of the novel gene gains, with the guinea-margaritiferum accessions possessing the most unique novel genes within the cultivated S. bicolor lines (4.8%; Supplementary Fig. S49 ; Supplementary Data 16 ). The possession of novel genes, together with the depth of sequence variations specific to the guinea-margaritiferum genotypes, highlights the potential untapped diversity that exists within these accessions. As a staple food for 500 million resource-poor people in marginal environments and a model for other important crops, sorghum holds vital genetic resources as humanity confronts the nexus of food crisis and climate change. This study provides an unmatched resource to respond to these challenges by identifying a large high-quality SNP and indel data set in diverse sorghum genotypes. It includes the first sequences for Sorghum bicolor subsp. verticilliflorum , S. bicolor subsp . drummondii , the guinea-margaritiferum group and S. propinquum . We have identified that sorghum possesses a diverse primary gene pool but with decreased diversity in both landrace and improved groups. The guinea-margaritiferum group is confirmed as a second, more recent, domestication event, questioning its status within subspecies bicolor . The possession of new genes, a high frequency of novel SNPs and domestication features suggest the guinea-margaritiferums, in combination with S. bicolor subsp. verticilliflorum , subsp. drummondii and S. propinquum , provide an excellent source of diversity for sorghum improvement. In addition to providing a broad sample of the diversity in S. bicolor , the genotypes included in this study are known to display agronomically important traits including stay-green drought resistance, insect resistance, grain size and grain quality. The majority of these genotypes are parental lines of a recently developed sorghum Nested Association Mapping population [47] . Together these resources will facilitate the dissection of complex traits and the identification and exploitation of SNPs associated with favourable variants. This knowledge will maximise the contribution of C 4 grasses to the food security of the world’s most vulnerable and more efficient feed and fuel production. Resequencing and variant identification Total genomic DNA from 44 sorghum genotypes was extracted as described by Diversity Arrays Technology for Illumina sequencing. Paired-end sequencing libraries with insert sizes of 500 bp were constructed according to the manufacturer’s instructions, for sequencing on the HiSeq 2,000 platform. Paired-end reads (clean reads) obtained from sequencing were mapped in the sorghum BTx623 genome [6] with BWA software [13] . The detailed parameters used were as follows: ‘bwa aln –m 200000 –o 1 –e 50 –i 15 –L –I –t 4 –n 0.04 –R 30 -f’ ‘bwa sampe –a 650 –n 30 –N 30’ SAMtools [13] was used to convert mapping results to bam format. The bam alignments were then converted to pileup and glf formats using the pileup command. SNPs were then detected in three steps; First, realSFS [26] was used to identify SNPs in groups (three groups were defined, detailed in Supplementary Table S1 ; wild and weedy group, n =7; landrace group, n =18; and improved inbreds group, n =17) based on the Bayesian estimation of site frequency at every site. Sites with a probability to be variant >0.99 were further extracted to identify the putative SNP based on the following criteria; copy number ≤1.5, sequencing depth according to average depth of each accession, 100≤sequencing depth≤1,300, and distance of SNPs, the SNPs had to be a minimum of 5 bp apart, with the exception of minor allele frequencies (MAF ≥0.05) where SNPs were retained when the distance between SNPs was less than 5 bp. In this procedure, a total of 15,564,426 raw population SNPs were identified, which were further filtered to 6,873,194 when the additional filtering criteria were applied. Second, SOAPsnp [48] was used to calculate the likelihood of genotypes of each individual. In each individual, SNPs were filtered by the quality value (≥20), the minimum number of required reads supporting each SNP (≥4), the maximum overall depth (≤100), the maximum copy number of flanking sequences (≤1.5) and the P value of the rank-sum test ( P >0.05). Third, the final SNP set was obtained by combining the two sets of possible SNPs above; 4,946,038 were identified as SNPs in both SNP sets with a missing data rate of less than 50% in the populations. To detect insertions and deletions, the Dindel pipeline [49] that uses a realignment algorithm was used, with the default parameters. Identification of regions identical-by-descent Regions that were expected to be identical-by-descent (IBD) between genotypes were masked before some analyses ( Supplementary Data 17 ). These regions were identified using pairwise SNP density comparisons and looking for contiguous 10 kb windows with low SNP density between samples. To be considered IBD, at least 100 consecutive 10 kb windows must have pairwise SNP densities of 25 or less at an average read depth of ten or more. A single window within the 100-window blocks was permitted to exceed the minimum number of SNPs and regions were assessed using a sliding window approach. Once individual blocks meeting these criteria were identified, overlapping features were merged and a consensus set of coordinates was extracted from regions common to all genotypes in the IBD analysis. Copy number variation A modified version of the recently described event-wise testing algorithm [20] was used to identify copy number variations. Read depth per 100 bp window was computed using this modified software, which adjusts for bias in read depth caused by GC content. SNP and indel validation SNP calling accuracy in addition to predicted base positions were validated utilizing Sanger sequencing and whole genome de novo assembly. Indel validation was determined via Sanger sequencing only. Sanger reads were aligned to the reference genome by BLAST software with only the best hit alignment used. All mismatch positions were recorded as SNPs. Likewise, predicted base positions that matched Sanger sequencing reads were also recorded as another measure of sequencing accuracy. The same alignments generated using BLAST software were used for indel calling; however, rather than mismatch sequences being analyzed, the gap positions were extracted. In total, 2,917 genotype-predicted base positions were detected, two of which were resequencing error. This equated to a genotype calling accuracy of 99.93%. Among the 2,917 base positions, 660 SNPs were identified, 1 of which was shown to be the result of sequencing error. Hence, SNP calling accuracy was 99.85% ( Supplementary Table S2a ). After data filtering using the Dindel pipeline, indels matching Sanger sequence equated to 42. Only a single indel was recorded as being erroneous, resulting in an indel calling accuracy of 97.62% ( Supplementary Table S2b ). Further validation of SNP calling accuracy was completed by comparing whole genome de novo assembly of two samples, S. bicolor subsp. verticilliflorum (PI300119) and S. propinquum 369-1 (both with sequencing depth > × 40) with their resequenced counterparts. Both genomes were assembled using SOAPdenovo [50] (K-mer=41). Only sequences (scaffold and contig) with length ≥1,000 bp and without N bases were retained. For genotypes PI300119 and S. propinquum 369-1, comparing the common position resequencing SNPs (≈0.72 and 1.27 M, respectively) with de novo data, we identified the same percentages (99.76% and 99.68%, respectively) ( Supplementary Table S3 ). Analysis of duplicate genes Annotated genes of S. bicolor were downloaded from the JGI website and a self-to-self BLAST performed. The four-fold degenerate transversion (4DTv) ratio was calculated for each best hit. The distribution of the 4DTv ratio of all gene pairs indicated that gene pairs in which both genes had a 4DTv ratio lower than 0.497 were recently duplicated, in agreement with previous studies [6] . Population genetics analysis SNPs were used to calculate the genetic distance between individuals. The neighbour-joining tree was constructed with treebest under the p -distances model, with bootstrapping (1,000). The software MEGA5 (ref. 51 ) was used for visualizing the phylogenetic tree. Principal component analysis of the SNPs was performed using the software EIGENSOFT [52] . The population structure was determined using the software FRAPPE [53] , we set MaxIter (Maximum iteration) parameter to 10,000, and the number of clusters ( K ) was considered from 2 to 12. The average pairwise divergence within a group ( θπ ) and the Watterson’s estimator ( θw ) were estimated for the whole genome of the three groups. A non-overlapping window size of 10 kb was used to estimate θπ , θw and Tajima’s D across the whole genome, in addition to a per FGS gene model basis (CDS, mRNA, intron, gene, 5′ UTR, 3′ UTR per predicted gene model). In each window, these parameters were calculated using a BioPerl module and an in-house perl script. F ST was calculated, based on the same windows, to measure population differentiation using another BioPerl module. Calculation of LD Correlation coefficient values ( r 2 ) of alleles were calculated using Haploview [54] to measure the LD level in the three populations. The parameters were set as follows: -dprime -minMAF 0.1 -hwcutoff 0.001 -memory 2000 -maxdistance 1000. The average r 2 value was calculated for each length of distance and LD decay figures were drawn using an R script [55] for the three groups of sorghum genotypes. Identification of novel genes Unmapped reads from each sample were assembled into contigs using SOAPdenovo [50] (default parameters). Assembled contigs for each sample were then filtered based on two criteria: (i) contigs <2 kb were excluded and (ii) redundant sequences were excluded based on a self-alignment approach. In total, 4,768 contigs with a total length of 20.8 Mb were identified and used as queries against the reference genome. Altogether, 808 (17%) of the contigs had coverage >30% and identify >80% with BTx623. The remaining 3,960 contigs were considered to be either real novel sequences or located in non-assembled heterochromatic regions. The GC ratio of the 20.8 Mb sequences was 41.4%, comparable to the GC ratio of the whole genome (41.4%). De novo gene annotation was conducted using the software AUGUSTUS [56] . Only one copy of the genes with more than 90% identity and 90% coverage by BLAT was retained. In total, 276 candidate novel genes were annotated. BLASTP was then used to compare the candidate novel genes against the NCBI nr database (high-quality hits ≥60% identity and 60% coverage). Identification of gene loss events Gene loss events were identified using read depth at 100 bp resolution from all predicted Sbicolor_79 gene models across all genotypes. In addition to the sequence bound by the gene models, 1 kb (10 windows) upstream and downstream of the annotated gene boundaries were used as reference read depths for each gene. A minimum average read depth of 10 was required for the flanking regions to assess deletions within genes. Large deletions of at least 50% of the annotated gene sequence in a single block were identified by comparing the read depth of consecutive windows within the genic regions to the average read depth of the 1 kb flanking sequences. Genic windows with less than 1% of the average read depth of the flanking windows were treated as putative deletions and gene deletions were identified by grouping consecutive windows meeting these criteria into single blocks that exceeded 50% of the total gene length. Identification of candidate genes under selection Regions of the genome under purifying selection are expected to have a lower diversity and reduced allele frequency in the descendant population compared with the same region in the ancestral population. The FGS gene-based population genetics summary statistics ( θπ , θw , Tajima’s D and F ST ) were used to identify candidate genes in the following three population pairwise comparisons: first, wild and weedy versus landraces to identify domestication events; second, landraces versus improved inbreds to identify improvement events; and third, wild and weedy versus improved inbreds to identify both domestication and improvement events. The following criteria were used to identify candidate genes in each of the three pairwise comparisons; F ST values ≥95% of population pairwise distribution; θπ and θw higher in ancestral population and ≤10% of descendant population distribution; negative Tajima’s D values in descendant population. In total, 772 unique candidate genes under purifying selection were identified across all three pairwise comparisons: 396 candidate domestication genes based on the wild and weedy versus landraces comparison, 251 candidate improvement genes based on the landraces versus improved inbreds comparison and 324 candidate domestication and/or improvement genes based on the wild and weedy versus improved inbreds comparison. A subset of 422 of these candidate genes under selection were used as input, together with 38 neutral genes, for the mlHKA test [31] for validation purposes. The MLHKA program was run under a neutral model, where numselectedloci=0, and then under a selection model, where numselectedloci>0. Significance was assessed by the mean log likelihood ratio test statistic, where twice the difference in log likelihood between the models is approximately chi-squared distributed with df equal to the difference in the number of parameters. GO-SLIM categories [44] were used to assess gene family enrichment across subsets of genes under selection and invariant genes. Accession codes: The sequencing data have been deposited in the NCBI Short Read Archive under accession codes SRS378430 to SRS378473 . How to cite this article: Mace, E. S. et al . Whole-genome sequencing reveals untapped genetic potential in Africa’s indigenous cereal crop sorghum. Nat. Commun. 4:2320 doi: 10.1038/ncomms3320 (2013).